High-efficiency organic light-emitting diodes with fluorescent emitters Fluorescence-based organic light-emitting diodes have continued to attract interest because of their long operational lifetimes, high colour purity of electroluminescence and potential to be manufactured at low cost in next-generation full-colour display and lighting applications. In fluorescent molecules, however, the exciton production efficiency is limited to 25% due to the deactivation of triplet excitons. Here we report fluorescence-based organic light-emitting diodes that realize external quantum efficiencies as high as 13.4–18% for blue, green, yellow and red emission, indicating that the exciton production efficiency reached nearly 100%. The high performance is enabled by utilization of thermally activated delayed fluorescence molecules as assistant dopants that permit efficient transfer of all electrically generated singlet and triplet excitons from the assistant dopants to the fluorescent emitters. Organic light-emitting diodes employing this exciton harvesting process provide freedom for the selection of emitters from a wide variety of conventional fluorescent molecules. Spin statistics states that one singlet exciton is generated for every three triplet excitons after the recombination of holes and electrons in organic semiconductor materials [1] . Light emission can be extracted through fluorescence or phosphorescence by the decay of these excitons from a singlet (S 1 ) or triplet (T 1 ) excited state to a ground state. By utilizing efficient radiative decay of electrically generated excitons, organic light-emitting diodes (OLEDs) are attracting intense attention for use as advanced displays and lighting sources. The external electroluminescence (EL) quantum efficiency ( η EQE ) of OLEDs is a key parameter and is described by the well-known equation where η int is the internal EL quantum efficiency and η out is the light-out-coupling efficiency. According to equation (1), η int is limited by the following three factors: (i) charge balance of injected holes and electrons ( γ ), (ii) efficiency of radiative exciton production ( η γ ) and (iii) photoluminescence (PL) quantum yield of the emitter molecules ( Φ PL ). The ideal γ can be achieved by circumspect design of OLED structures with the appropriate selection of charge transport layers, host–guest system, and anode and cathode materials. In addition, based on a proper molecular design for light emission, Φ PL of nearly 100% has been demonstrated in a wide variety of fluorescent and phosphorescent materials. However, η γ can severely limit η int if the 75% of electrically generated excitons formed in triplet states are not harvested. Several routes have been proposed to obtain a high η int through the efficient harvesting of triplet excitons in OLEDs. While the very first trials of ketone derivatives showing intense phosphorescence at low temperature opened a new method for triplet harvesting, the η EQE was limited to a low value [2] . Rare metal complexes containing Eu and Tb established intramolecular cascade energy transfer as another route to harvest triplet excitons but did not show promising η EQE [3] , [4] , [5] . Later, a successful strategy was realized using room temperature phosphorescent emitters such as platinum and iridium complexes. In this case, according to the mixing of the spin orbitals of S 1 and T 1 states due to the presence of a heavy atom, the radiative decay rate from a T 1 state to a ground state is significantly accelerated, resulting in the radiative decay of nearly 100% of triplet excitons [6] , [7] , [8] , [9] , [10] . In addition, the utilization of phosphorescence emitters as a triplet sensitizer has been proposed [11] , [12] . Using this process, triplet harvesting realized by energy transfer from the T 1 state of a phosphorescent emitter such as an iridium 2-phenylpyridine complex to the S 1 state of a fluorescent emitter via dipole–dipole coupling (that is, Förster energy transfer, FRET) resulted in an η int of ~45% (ref. 12 ). However, the rather limited η int is due to the presence of the competitive deactivation process of triplet–triplet energy transfer. Although OLEDs based on fluorescent molecules, which are composed of simple aromatic compounds, have continued to attract interest because of their longer operational lifetimes in blue OLEDs, higher colour purity (narrow spectral width) EL and broader freedom of molecular design compared with phosphorescence-based OLEDs [13] , [14] , [15] , the η int of traditional fluorescence-based OLEDs is limited to less than 25% even in the ideal case. Therefore, the enhancement of η int in OLEDs using conventional fluorescence-based emitters is still obviously a major concern for the development of future OLEDs. To achieve this, singlet exciton generation via a triplet–triplet annihilation (TTA) process is one possible route [16] , [17] . However, the theoretical upper limit of the singlet exciton production ratio when the TTA process is included is still less than 62.5%, corresponding to an η EQE of 12.5% in the ideal case [18] . Recently, we demonstrated an alternative route for increasing η int by using a thermally activated delayed fluorescence (TADF) process [19] , [20] , [21] , [22] , [23] . In the TADF process, light emission can be extracted as delayed fluorescence after intersystem crossing (ISC) from the T 1 to the S 1 states in TADF emitters, resulting in efficient radiative decay from the S 1 state. In fact, after comprehensive development of TADF materials, an η int of nearly 100% was realized in green OLEDs [21] . In addition to the use of the TADF process for emitters in OLEDs, we propose a promising route for triplet harvesting by applying TADF molecules as an assistant dopant in OLEDs. Thus, the OLED is composed of a double-dopant system—that is, a wide-energy-gap host, a TADF-assistant dopant and a fluorescent emitter dopant—that leads to η γ =100%. In this system, triplet excitons created on an assistant TADF molecule ( ) by electrical excitation are upconverted to the S 1 state of the TADF molecule ( ), and all excitons are transferred to the S 1 state of a fluorescent emitter molecule ( ) via a FRET process, which results in efficient radiative decay from of the fluorescent emitter. On the basis of this cascade energy transfer, we demonstrate highly efficient OLEDs with η EQE as high as 13.5, 15.8, 18 and 17.5% for blue, green, yellow and red colours, respectively. We use the TADF molecules 10-phenyl-10H, 10′H-spiro[acridine-9,9′-anthracen]-10′-one (ACRSA) [23] , 3-(9,9-dimethylacridin-10(9H)-yl)-9H-xanthen-9-one (ACRXTN), 2-phenoxazine-4,6-diphenyl-1,3,5-triazine (PXZ-TRX) [20] and 2,4,6-tri(4-(10H-phenoxazin-10H-yl)phenyl)-1,3,5-triazine (tri-PXZ-TRZ) [22] as assistant dopants and 2,5,8,11-tetra-tert-butylperylene (TBPe), 9,10-Bis[N,N-di-(p-tolyl)-amino]anthracene (TTPA), 2,8-di-tert-butyl-5,11-bis(4-tert-butylphenyl)-6,12-diphenyltetracene (TBRb) and tetraphenyldibenzoperiflanthene (DBP) as fluorescent emitter dopants ( Fig. 1a ). These fluorescent molecules have been widely used as conventional fluorescent emitters in OLEDs and are commercially available [24] , [25] , [26] , [27] . As host materials, we use bis-(2-(diphenylphosphino)phenyl)ether oxide (DPEPO), 1,3-Bis(N-carbazolyl)benzene (mCP), 3,3-di(9H-carbazol-9-yl)biphenyl (mCBP) and 4,4′-bis(9-carbazolyl)-1,1′-biphenyl (CBP) for the blue, green, yellow and red OLEDs, respectively. In this double-dopant system, the assistant dopant does not itself emit light but passes all of the electrically generated excitons to fluorescent emitter molecules for radiative decay. 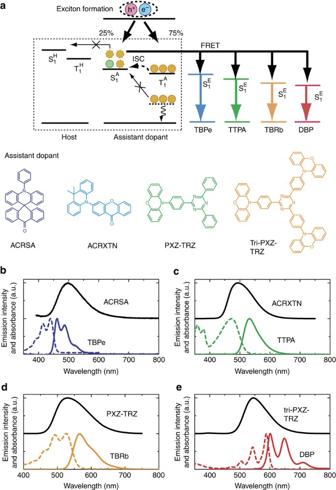Figure 1: Energy transfer mechanism. (a) Schematic illustration of proposed energy transfer mechanism in the emitter dopant:assistant dopant:host matrix under electrical excitation and chemical structures of the assistant dopants used in this study. (b–e) Fluorescence spectra of assistant dopant:host co-deposited film (upper), and absorption (dashed line) and fluorescence (solid line) spectra of emitter dopant in solution (10−5mol l−1in CH2Cl2) (bottom). Rather large Förster transfer radii of ~2.2, ~7.3, ~6.9 and ~10 nm were estimated for blue, green, yellow and red EML matrices based on the spectral overlap between the absorption spectrum of the acceptor and the PL spectrum of the donor, suggesting that efficient FRET is possible. Figure 1: Energy transfer mechanism. ( a ) Schematic illustration of proposed energy transfer mechanism in the emitter dopant:assistant dopant:host matrix under electrical excitation and chemical structures of the assistant dopants used in this study. ( b – e ) Fluorescence spectra of assistant dopant:host co-deposited film (upper), and absorption (dashed line) and fluorescence (solid line) spectra of emitter dopant in solution (10 −5 mol l −1 in CH 2 Cl 2 ) (bottom). Rather large Förster transfer radii of ~2.2, ~7.3, ~6.9 and ~10 nm were estimated for blue, green, yellow and red EML matrices based on the spectral overlap between the absorption spectrum of the acceptor and the PL spectrum of the donor, suggesting that efficient FRET is possible. Full size image Energy transfer process Figure 1a shows an energy transfer diagram for the emitter layers (EMLs) in our cascade-type EL devices. The emitter and assistant dopant molecule combinations and concentrations studied as EMLs here are listed in Table 1 . In the case of an EML without any assistant dopant, the injected carriers are transported on the host molecules, and the carriers are eventually trapped on an emitter dopant due to its shallower highest occupied molecular orbital and deeper lowest unoccupied molecular orbital compared with those of the host material. This results in direct carrier recombination dominantly on the emitter dopants. Therefore, no triplet excitons contribute to the total EL efficiency. Table 1 Components of the emitter layers of the four colour OLEDs. Full size table On the other hand, when assistant dopants are doped into these EMLs, exciton formation mainly on the assistant molecules is desired. Here to reduce the effect of direct carrier trapping on the emitter molecules in the EMLs, the doping concentration of the emitter dopants was held at 1 wt%. Conversely, assistant dopants were doped into the EMLs in doping concentrations ranging between 15 and 50 wt%, which ensures that the assistant dopants act as the main carrier recombination centres in the EMLs. Thus, after both singlet ( ) and triplet ( ) exciton formation on the assistant dopants, the formed triplet excitons are upconverted to the state through ISC because of the rather small energy gap between the and levels (Δ E ST ), as summarized in Table 1 . Then, according to the spectral overlap between the absorption spectra of the emitter molecules and the PL spectra of the assistant dopants ( Fig. 1b–e ), the exciton energies are resonantly transferred to the states of emitter molecules based on a FRET process. Finally, light can be emitted as delayed fluorescence from the state of the emitter molecules. If conventional fluorescence molecules were used as the assistant dopant, triplet excitons would non-radiatively decay from to the ground state and would not contribute to light emission because of the large Δ E ST of conventional fluorescence molecules as shown in Fig. 1a . Thus, the created triplet excitons would not contribute to the energy transfer processes if the assistant dopant is a conventional fluorescence material. The proposed influence of concentration on carrier trapping and recombination is well supported by the dependence of η EQE on the concentration of the assistant dopant as shown in Supplementary Figs 1–3 and Supplementary Note 1 . Here we observed the best η EQE -luminance ( L ) characteristics with the assistant dopant concentration of 15%. In the case of assistant dopant concentrations less than 15%, carrier recombination may not perfectly occur on the assistant dopants, while Dexter energy transfer from the assistant dopants to the triplet level of a fluorescent emitter ( ) or concentration quenching of the assistant dopants may happen in the case of the concentrations over 15%. The optimum concentration would change for different combinations of host and guest molecules having different carrier transport and photophysical characteristics. We note that the host layers have both higher singlet ( ) and triplet ( ) energy levels than those of the assistant molecules, and . Therefore, back energy transfer from the state of the assistant dopants to the state of the host layers is inhibited. In addition, dispersing the assistant dopants in a host matrix can additionally prevent direct energy transfer from to —that is, minimize a Dexter energy transfer process that would result in losses [11] . OLED characteristics On the basis of the optimized configuration of EMLs for blue, green, yellow and red EL, full-colour OLEDs were fabricated to demonstrate the impact of this triplet harvesting process on OLED performance. The η EQE - L curves of the four OLEDs are shown in Fig. 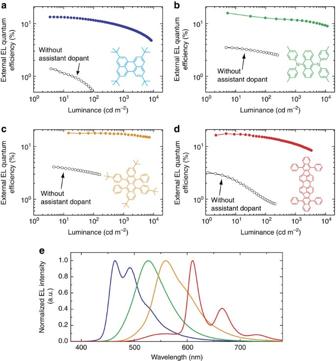Figure 2: Device performance of OLEDs. (a–d) External EL quantum efficiency as a function of luminance for the blue, green, yellow and red OLEDs. The external EL quantum efficiency for OLEDs without an assistant dopant is plotted as open symbols. Inset: chemical structures of emitter dopants used in this study. (e) EL spectra of the devices at a luminance of 100 cd m−2. 2a–d , and Table 2 summarizes their device performance. Although the OLEDs without assistant dopants, which use only conventional single doping by fluorescent dopants, show low device performance as shown by the open circles ( η EQE <5%), remarkably high η EQE of 13.4, 15.8, 18 and 17.5% for blue, green, yellow and red EL were achieved by including the assistant dopants. In addition, the magnitudes of the slopes of the η EQE - L curves of the double-dopant systems are much lower than those of the corresponding single-dopant systems at similar luminance, indicating that the efficiency roll-off characteristics are well suppressed in the double-dopant system. The reduced roll-off is probably because of the expansion of the carrier recombination site or the reduction of the interaction between excitons and polarons (that is, exciton–polaron annihilation) as a result of rapid energy transfer from the carrier recombination centre (TADF assistant dopants) to the emission centre (fluorescent emitter dopants). Figure 2: Device performance of OLEDs. ( a – d ) External EL quantum efficiency as a function of luminance for the blue, green, yellow and red OLEDs. The external EL quantum efficiency for OLEDs without an assistant dopant is plotted as open symbols. Inset: chemical structures of emitter dopants used in this study. ( e ) EL spectra of the devices at a luminance of 100 cd m −2 . Full size image Table 2 Device performance of the four colour OLEDs with assistant dopants for triplet harvesting. Full size table The EL spectra of the OLEDs are presented in Fig. 2e , Supplementary Fig. 4 and Supplementary Note 2 . These OLEDs emit a full range of visible colours from blue (462 nm) to red (610 nm). Although a weak emission originating from the assistant dopant is observed in the red OLED, other OLEDs showed pure emission originating from the emitter dopants that is in good accordance with the PL spectrum of the emitter dopants in solution. Here Φ PL of 80±2, 81±2, 90±2 and 88±2% were obtained for the blue, green, yellow and red emitter dopants when doped with assistant dopants in films ( Table 1 ). Thus, we can estimate η γ of 55–84%, 65–97%, 66–100% and 66–99%, respectively, assuming a charge carrier balance factor of 1 and a light-out-coupling efficiency of 20–30% (refs 28 , 29 ). These results clearly indicate that the devices overcame the theoretical limit of 25% for the singlet exciton production efficiency that is assumed for fluorescence-based OLEDs and even that of 62.5% in the case of TTA [18] . 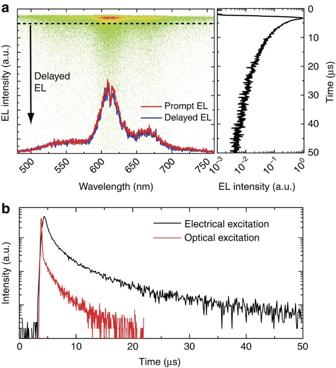Figure 3: Transient EL characteristics. (a) Time-resolved electroluminescence image for the red OLED. The streak image (left) and time-resolved EL decay curve (right) are for the red OLED under electrical excitation with a pulse of 1 μs at 300 K. A delayed EL spectrum was collected from 3 to 50 μs after excitation. (b) Time-resolved PL and EL response of a 1 wt%-DBP:15 wt%-tri-PXZ-TRZ:CBP film (red line) and 1 wt%-DBP:15 wt%-tri-PXZ-TRZ:CBP-based OLED (black line), respectively. Transient EL analysis In order to confirm the contribution of singlet exciton generation via energy transfer from the assistant dopants to the emitter dopants after harvesting triplet excitons on the assistant dopants under electrical excitation, transient EL was measured with an electrical excitation pulse width of 1 μs at 300 K. Figure 3a shows the streak image and the transient EL decay curve obtained from the red OLED with an EML of 1 wt% DBP and 15 wt% tri-PXZ-TRZ in a CBP host matrix. After turning off the electrical pulse excitation, a clear delayed component with emission bands centred at 610 nm was observed. In addition, the emission spectrum of the delayed fluorescence is consistent with that of the prompt component, which is consistent with the described mechanism of triplet to singlet exciton upconversion in tri-PXZ-TRZ followed by successive resonant singlet energy transfer to the states of DBP emitters. Figure 3: Transient EL characteristics. ( a ) Time-resolved electroluminescence image for the red OLED. The streak image (left) and time-resolved EL decay curve (right) are for the red OLED under electrical excitation with a pulse of 1 μs at 300 K. A delayed EL spectrum was collected from 3 to 50 μs after excitation. ( b ) Time-resolved PL and EL response of a 1 wt%-DBP:15 wt%-tri-PXZ-TRZ:CBP film (red line) and 1 wt%-DBP:15 wt%-tri-PXZ-TRZ:CBP-based OLED (black line), respectively. Full size image Here we describe the exciton formation process in the double-dopant system under either optical or electrical excitation. In the case of optical excitation, singlet excitons are mainly generated in the state of a CBP host molecule by photoabsorption, and nearly all of the singlets are then resonantly transferred to the state of tri-PXZ-TRZ molecules because of the large concentration of the assistant dopants. In addition, a number of singlet excitons in tri-PXZ-TRZ would also be formed by direct absorption. Next, a fraction of the singlet excitons is transferred into the state of DBP through a FRET process, producing the prompt fluorescence decay of DBP. Simultaneously, singlet excitons on tri-PXZ-TRZ also decay to the state internally through ICS and are successively upconverted into the state again by thermal conversion, followed by energy transfer via FRET to the state of DBP that produces the delayed emission. Here we can ignore the direct formation of excitons on DBP because of the dilute concentration of 1 wt%. Under electrical excitation, on the other hand, since the singlet and triplet excitons are directly created on the and states of the tri-PXZ-TRZ molecules based on the exciton branching ratio of 25–75%, respectively, the contribution of the delayed fluorescence in the total emission is significantly larger compared with that of the optical excitation, as shown in Fig. 3b . Device operational stability The introduction of assistant dopants into a host–guest system provides not only a significant enhancement of η EQE but also an enhancement of device operational stability under electrical excitation. For example, the normalized luminance of the yellow OLEDs as a function of operation time at a constant current density of 10 mA cm −2 are presented in Fig. 4 . Although a rapid decrease in luminance was observed in the OLED without assistant dopants (device B), the OLED with the assistant dopants (device A) showed improved luminance decay characteristics compared with that of the OLED without the assistant dopants, resulting in an improved operational lifetime, defined as the elapsed operation time at which the luminance drops to 50% of the initial value, of 194 h. The driving voltages of the devices are also rather stable, displaying a rise of less than 0.5 V after 100 h of operation. More interestingly, the operational lifetime was longer than that of the OLED with PXZ-TRZ molecules as the emitter dopant (device C) while the voltage rise curves are almost the same, indicating that the combination of fluorescent emitter dopants and TADF assistant dopants provides improved device performance. We note that the nearly identical film morphology for each of the co-deposited films compared with that of the host-only films suggests that device stability is not influenced by a morphology change caused by the dopant molecules as shown in Supplementary Fig. 5 and Supplementary Note 3 . Since it is well established that TBRb is a stable emitter electrochemically [26] , the differences in reliability would be because of the change of carrier recombination and exciton formation area with and without the presence of the assistant dopants, in addition to the electrochemical stability of emitter molecules. 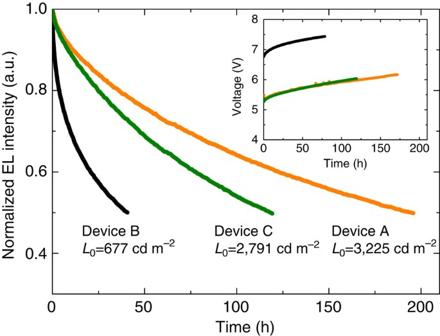Figure 4: Device stability of yellow OLEDs. For operational lifetime measurement of the double-dopant system, an OLED with a device structure of ITO/α-NPD (35 nm)/1 wt%-TBRb:25 wt%-PXZ-TRZ:mCBP (30 nm)/T2T (10 nm)/Alq3(55 nm)/LiF (0.8 nm)/Al (100 nm) (device A) was used. To confirm the effect of the assistant dopant, OLEDs with an EML of either 1 wt%-TBRb:mCBP (device B) or 25 wt%-PXZ-TRZ:mCBP (device C) were also measured at a constant current density of 10 mA cm−2. Initial luminances (L0) are 3,225, 677 and 2,791 cd m−2for devices A, B and C, respectively. Inset: voltage rise curves for devices A, B and C (coloured accordingly). Figure 4: Device stability of yellow OLEDs. For operational lifetime measurement of the double-dopant system, an OLED with a device structure of ITO/α-NPD (35 nm)/1 wt%-TBRb:25 wt%-PXZ-TRZ:mCBP (30 nm)/T2T (10 nm)/Alq 3 (55 nm)/LiF (0.8 nm)/Al (100 nm) (device A) was used. To confirm the effect of the assistant dopant, OLEDs with an EML of either 1 wt%-TBRb:mCBP (device B) or 25 wt%-PXZ-TRZ:mCBP (device C) were also measured at a constant current density of 10 mA cm −2 . Initial luminances ( L 0 ) are 3,225, 677 and 2,791 cd m −2 for devices A, B and C, respectively. Inset: voltage rise curves for devices A, B and C (coloured accordingly). Full size image Our results suggest that both a higher η EQE and an enhancement of operational stability can be expected with an optimum EML design using a wide variety of TADF and fluorescent materials. As numerous electrochemically stable fluorescent emitters have been widely developed in the past two decades, the triplet harvesting mechanism realized here can provide a greater flexibility in the design of OLED architectures. In addition, since η out can exceed 20% by using emitter molecules with horizontally oriented dipoles [30] , the flexibility of simple aromatic compound design can further boost the η EQE by enhancement of η out without special light-out-coupling structures. In summary, we presume that the cascade energy transfer scheme using TADF assistant dopants and fluorescent emitter dopants will be the most promising device architecture for OLEDs with ultimate performance. Materials mCP, 4,4′-cyclohexylidenebis[N,N-bis(4-methylphenyl)benzenamine] (TAPC), 2,2′,2′′-(1,3,5-benzinetriyl)-tris(1-phenyl-1-H-benzimidazole (TPBi), TBPe, TTPA, TBRb and DBP were purchased from Luminescence Technology Corp. mCBP was purchased from NARD Institute Ltd. CBP, 4,4′-bis(N-phenyl-1-naphthylamino)biphenyl (α-NPB) and tris(8-hydroxyquinolinato)aluminum (Alq3) were used as received from the Nippon Steel Chemical Co., Ltd. ACRSA, DPEPO [31] , 2-phenoxazine-4,6-diphenyl-1,3,5-triazine (PXZ-TRX), tri-PXZ-TRZ and 2,4,6-tris(biphenyl-3-yl)-1,3,5-triazine (T2T) [32] were synthesized according to the reported procedures. Synthesis of ACRXTN We synthesized ACRXTN according to the general procedure. The complete synthetic route for ACRXTN and the 1H NMR spectrum of ACRXTN are included in the Supplementary Methods section and Supplementary Fig. 6 , respectively. NMR spectra were obtained with a Bruker Biospin Avance-III 500 NMR spectrometer at ambient temperature. High-resolution mass spectrometry by fast atom bombardment was performed using a JEOL JMS-700 spectrometer. 3-bromo-9H-xanthen-9-one 1.38 g (5 mmol), 9,9-dimethyl-9,10-dihydroacridine 1.15 g (5.5 mmol), tert-BuONa 0.96 g (10 mmol), tri-tert-butylphosphonium tetrafluoroborate 145 mg (0.5 mmol) and palladium acetate 56 mg (0.25 mmol) were put into a flask and purged three times by nitrogen/vacuum cycle. Then, anhydrous toluene was added and refluxed for 8 h. After cooling to room temperature, the resulting solution was filtered through celite and concentrated. The crude product was purified using a silica gel chromatography (CH 2 Cl 2 :hexane= 8:2) and recrystallized twice from mixed solvent of hexane:AcOEt =9:1 ml g −1 . The desired product was obtained as yellow powder (2.06 g, 85%). 1 H-NMR (500 MHz, CDCl 3 ): δ (p.p.m. )=8.53 (d, 1H, 8.5 Hz), 8.38 (dd, 1H, 8 Hz), 7.74 (ddd, 1H, 8.6, 7.2, 1.8 Hz), 7.53 (d, 1H, 1.9 Hz), 7.52–7.46 (m, 3H), 7.42 (ddd, 1H, 8.1, 7.2, 1 Hz), 7.38 (dd, 1H, 8.5, 2 Hz), 7.08–6.98 (m, 4H), 6.53 (dd, 2H, 7.8, 1.6 Hz). 13 C-NMR (125 MHz, CDCl 3 ): δ (p.p.m. )=176.47, 157.83, 156.25, 148.09, 140.28, 134.94, 132.55, 129.32, 126.79, 126.45, 125.27, 124.59, 124.20, 121.99, 121.96, 120.52, 117.95, 117.57, 115.88, 36.38, 30.53. High-resolution mass spectrometry (m/z): [M+H]+ calculated for C28H22NO2, 404.1651; found, 404.1651. Optical characterization of organic thin films PL quantum efficiency was measured by an absolute PL quantum yield measurement system (C11347-01, Hamamatsu Photonics) under the flow of nitrogen gas with an excitation wavelength of 337 nm. Low-temperature PL intensity and emission lifetimes were measured using a streak camera (C4334, Hamamatsu Photonics) and cryostat (Iwatani Industrial Gases Co.) with a nitrogen gas laser (MNL200, Laser Technik) as an excitation light source under a pressure of about 3 Pa. Fabrication of OLEDs Glass substrates with a pre-patterned, 100-nm-thick, 100 Ohm sq −2 tin-doped indium oxide (ITO) coating were used as anodes. Substrates were washed by sequential ultrasonication in neutral detergent, distilled water, acetone and isopropanol, and then exposed to ultraviolet–ozone (NL-UV253, Nippon Laser & Electronics Lab) to remove adsorbed organic species. After pre-cleaning of the substrates, effective device areas of 1 mm 2 were defined on the patterned-ITO substrates by a polyimide insulation layer using a conventional photolithography technique. Substrates were treated with ultraviolet–ozone for 25 min and immediately transferred into the evaporation chamber. Organic layers were formed by thermal evaporation. Doped emitting layers were deposited by co-evaporation. Deposition was performed under vacuum at pressures of <5 × 10 −5 Pa. Devices were exposed to nitrogen gas once after formation of the organic layers to apply a metal mask that defines the cathode area. After device fabrication, devices were immediately encapsulated with glass lids using epoxy glue in a nitrogen-filled glove box (O 2 <0.1 p.p.m., H 2 O<0.1 p.p.m.). Commercial calcium oxide desiccant (Dynic Co.) was included in each encapsulated package. Blue OLEDs with the structure ITO/α-NPB (35 nm)/mCP (10 nm)/1 wt%-TBPe: 15 wt%-ACRSA: DPEPO (15 nm)/DPEPO (8 nm)/TPBi (57 nm)/LiF (0.8 nm)/Al (100 nm) were fabricated. As a control device, an OLED with an EML that consisted of 1 wt%-TBPe: DPEPO was also made. Green OLEDs with the structure ITO/TAPC (35 nm)/1 wt%-TTPA: 50 wt%-ACRXTN: mCP (15 nm)/TPBi (65 nm)/LiF (0.8 nm)/Al (100 nm) were fabricated. As a control device, an OLED with an EML consisting of 1 wt%-TTPA: mCP was also made. Yellow OLEDs with the structure ITO/TAPC (35 nm)/1 wt%-TBRb:25 wt%-PXZ-TRX:mCBP (30 nm)/T2T (10 nm)/Alq 3 (55 nm)/LiF (0.8 nm)/Al (100 nm) were fabricated. As a control device, an OLED with an EML consisting of 1 wt%-TBRb: mCBP was also made. Red OLEDs with the structure ITO/TAPC (35 nm)/1 wt%-DBP:15 wt%-tri-PXZ-TRZ:CBP (15 nm)/TPBi (65 nm)/LiF (0.8 nm)/Al (100 nm) were fabricated. As a control device, an OLED with an EML consisting of 1 wt%-DBP: CBP was also made. Schematic diagrams of the energy levels of the fabricated devices and the chemical structures of the assistant dopant materials used in them are presented in Supplementary Fig. 7 . Characterization of OLEDs The current density–voltage–luminance characteristics of the OLEDs were evaluated using a source meter (Keithley 2400, Keithley Instruments Inc.) and an absolute external quantum efficiency measurement system (C9920-12, Hamamatsu Photonics). The OLEDs were mounted to the entrance port of the measurement system’s integrating sphere to collect the photons emitted from the front face of the devices. Each EL spectrum was collected by an optical fiber connected to a spectrometer (PMA-12, Hamamatsu Photonics). The repeatability of device performances of the present devices was confirmed by four different samples. To confirm the validity of our η EQE measurements, we also measured η EQE using another independent measurement system based on a luminance meter ( Supplementary Fig. 8 and Supplementary Note 4 ). Time-resolved EL decay curves were obtained using a streak camera (C4334, Hamamatsu Photonics) with a pulse generator (81101A, Agilent) as an electrical excitation source. The operational lifetime was measured using a luminance meter (SR-3AR, TOPCON) at a constant DC current. All measurements were performed in ambient atmosphere at room temperature. How to cite this article: Nakanotani, H. et al. High-efficiency organic light-emitting diodes with fluorescent emitters. Nat. Commun. 5:4016 doi: 10.1038/ncomms5016 (2014).